αTAT1 is the major α-tubulin acetyltransferase in mice Post-translational modification of tubulin serves as a powerful means for rapidly adjusting the functional diversity of microtubules. Acetylation of the ε-amino group of K40 in α-tubulin is one such modification that is highly conserved in ciliated organisms. Recently, αTAT1, a Gcn5-related N -acetyltransferase, was identified as an α-tubulin acetyltransferase in Tetrahymena and C . elegans . Here we generate mice with a targeted deletion of Atat1 to determine its function in mammals. Remarkably, we observe a loss of detectable K40 α-tubulin acetylation in these mice across multiple tissues and in cellular structures such as cilia and axons where acetylation is normally enriched. Mice are viable and develop normally, however, the absence of Atat1 impacts upon sperm motility and male mouse fertility, and increases microtubule stability. Thus, αTAT1 has a conserved function as the major α-tubulin acetyltransferase in ciliated organisms and has an important role in regulating subcellular specialization of subsets of microtubules. Microtubules are highly conserved polymerized dimers of α- and β-tubulin, with a broad range of functions in eukaryotic cells such as mitosis, intracellular transport, cellular morphology and motility of cilia [1] . The functional diversity of microtubules arises from a number of sources including interaction with microtubule-associated proteins, differential expression of genetically encoded tubulin isotypes and post-translational modification [2] . Of these, post-translational modification of tubulin may be particularly important in tuning the function of microtubules in organelles such as cilia and flagella [3] . Acetylation at the ε-amino group of K40 of α-tubulin is one such modification that was first described in the flagella of Chlamydomonas [4] , [5] . Acetylation of α-tubulin is especially enriched in primary and motile cilia [6] , and in neuronal axons [7] , and is used extensively as a marker of these structures. Accordingly, α-tubulin acetylation has been suggested to influence both the assembly and disassembly of the primary cilium [8] , [9] , and accelerate kinesin-mediated transport along microtubule tracks in axons [10] . Recently, a number of enzymes have been implicated in the regulation of microtubule acetylation including the deacetylases HDAC6 (ref. 11 ) and SirT2 (ref. 12 ), and the acetyltransferases ARD1-NAT1 (ref. 13 ), ELP3 (ref. 14 ), San [15] , GCN5 (ref. 16 ) and αTAT1 (refs 9 , 17 , 18 ). Of these, compelling evidence supports a role for αTAT1 as the major α-tubulin acetyltransferase in Tetrahymena and C. elegans [9] , [17] . Genetic ablation of aTAT1 genes in these organisms leads to an almost complete loss of α-tubulin acetylation. In Tetrahymena , this in turn slows the growth of cells treated with microtubule depolymerizing agents and increases the rate of depolymerization of axonemes [17] . In C. elegans , deletion of αTAT1 orthologues MEC17 and αTAT-2, reduces touch sensitivity [9] , [17] and disrupts microtubule structure and organization in touch receptor neurons [18] , [19] . Importantly, these effects depend upon both the acetyltransferase activity of α-TAT1 and on other as yet unknown functions of this protein [18] . The role of αTAT1 has been less extensively explored in vertebrates. In zebrafish, depletion of the Atat1 orthologue mec17 results in developmental defects such as reductions in body and head size, hydrocephalus and neuromuscular deficiencies [17] . Akin to mammals, acetylated microtubules in zebrafish are located principally in neurons and cilia [20] , [21] . Intriguingly, however, it has been reported that while zebrafish mec17 morphants display an almost complete loss of K40 α-tubulin acetylation in neurons, acetylation of α-tubulin in cilia is preserved [17] . This raises the question as to whether an additional acetyltransferase may be responsible for α-tubulin acetylation in vertebrate cilia. To determine whether αTAT1 functions as an α-tubulin acetyltransferase in mammals, we generated mice with a targeted deletion of Atat1. Strikingly, in homozygous Atat1 knockout mice (Atat1 −/− ) we were unable to detect tubulin acetylation in embryonic or adult mice across multiple tissues examined. Moreover, at the subcellular level, detectable tubulin acetylation was absent in both the cytoplasm and in cilia. We examined these structures in more detail and found that in the cytoplasm, deletion of Atat1 rendered microtubules more resistant to depolymerization. Primary cilia and motile cilia of the oviduct were, however, present in normal numbers and displayed no abnormalities in their morphology or length. At the whole animal level, Atat1 −/− mice were viable, developed normally and displayed no major behavioural phenotype. However, we detected a reduction in mean litter size from male homozygote breedings. In light of the striking absence of detectable acetylation in flagella we examined spermatozoa from these mice and observed deficits in their morphology and motility. Thus, αTAT1 is the major, if not the sole, α-tubulin acetyltransferase in mice and is required for normal sperm flagellar function. Generation of Atat1 −/− mice To explore the role of αTAT1 and microtubule acetylation in vivo in mammals, we generated Atat1 knockout mice. The Atat1 gene is located on chromosome 17 of the mouse genome and consists of 15 exons ( Fig. 1a ). All annotated protein-coding Atat1 splice variants have the first seven exons in common (ENSMUS accession code G00000024426) and exons 3–7 encode the acetyltransferase domain [22] , [23] , [24] , [25] . We therefore designed a targeting construct whereby exons 1–6 were flanked with loxp sites to enable Cre-mediated tissue-specific deletion. A floxed neomycin cassette was also introduced to enable selection of properly targeted ES cells ( Fig. 1b ). Positive ES cell clones were identified using southern hybridization, and chimeric mice were obtained that were crossed with Flp-expressing transgenic mice to remove the neomycin cassette (termed Atat1 fl/fl ). Subsequently, Atat1 −/− mice were generated by deleter -Cre-mediated [26] excision of the LoxP-flanked Atat1 fl/fl allele. Further crosses were undertaken to remove the Flp and Cre transgenes and experiments were performed on Atat1 −/− mice using Atat1 fl/fl as controls. Validation of this strategy was achieved using southern hybridization ( Fig. 1c ) and we were unable to detect Atat1 transcripts by RT–PCR in Atat1 −/− mice. Mice were routinely genotyped using PCR ( Fig. 1d ). Both Atat1 fl/fl and Atat1 −/− were viable and showed no obvious phenotype. 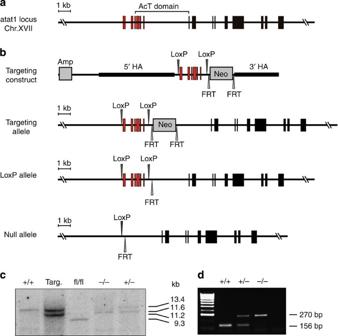Figure 1: Atat1 alleles. (a) Genomic locus of theAtat1gene. Black boxes indicate exons, red boxes indicated targeted exons. (b) Map of the pDTA-Atat1 targeting construct, targeting allele, LoxP allele and null allele. HA; homology arm,AmpandNeo; ampicillin (bacterial) and neomycin (mammalian) resistance genes. LoxP and FRT sites are indicated. (c) Southern blot analysis of genomic DNA for indicated genotypes. ‘kb’ indicates kilobases. (d) Genotyping PCR of the wild-type (+/+), heterozygous (+/−) and homozygous (−/−) knockouts. Figure 1: Atat1 alleles. ( a ) Genomic locus of the Atat1 gene. Black boxes indicate exons, red boxes indicated targeted exons. ( b ) Map of the pDTA-Atat1 targeting construct, targeting allele, LoxP allele and null allele. HA; homology arm, Amp and Neo ; ampicillin (bacterial) and neomycin (mammalian) resistance genes. LoxP and FRT sites are indicated. ( c ) Southern blot analysis of genomic DNA for indicated genotypes. ‘kb’ indicates kilobases. ( d ) Genotyping PCR of the wild-type (+/+), heterozygous (+/−) and homozygous (−/−) knockouts. Full size image Absence of K40 α-tubulin acetylation in Atat1 −/− mice To explore the consequence of Atat1 ablation, we first examined α-tubulin K40 acetylation in multiple adult tissues by immunoblotting with a well-characterized monoclonal antibody that recognizes acetylated K40 on α-tubulin (6-11b-1 (ref. 6 )). As shown in Fig. 2 and Supplementary Fig. S1a,b , α-tubulin acetylation is particularly prominent in nervous tissues and testes of control mice, with lower levels present in kidney, lung, ovary and spleen. Liver, pancreas and heart had barely detectable levels of α-tubulin K40 acetylation. Remarkably, in homozygous Atat1 knockout mice we were unable to detect K40 α-tubulin acetylation in the majority of tested tissues (for example, in the brain; Supplementary Fig. S1c ), although a very weak signal was evident in heart and liver ( Fig. 2b ). To further quantify α-tubulin acetylation during development we examined immunoblots of E12.5 embryos and embryonic fibroblasts and observed pronounced microtubule acetylation in control animals. Atat1 −/− embryos and fibroblasts, however, displayed a complete absence of detectable K40 α-tubulin acetylation ( Fig. 2c and Supplementary Fig. S1b ). We also investigated whether the lack of K40 α-tubulin acetylation might impact upon expression levels of α-tubulin. As shown in Fig. 2a–c , the total level of α-tubulin protein was not altered in knockout animals. 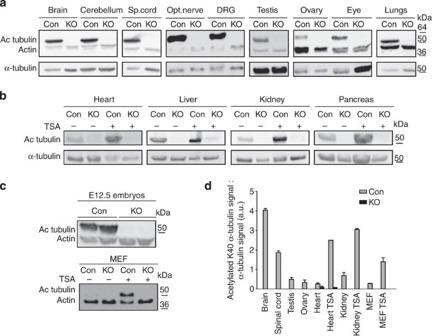Figure 2: Microtubule acetylation in Atat1−/−mice. (a) Absence of detectable α-tubulin K40 acetylation in Atat1−/−mice as determined by immunoblotting of tissues in adults. Total levels of α-tubulin are not changed in Atat1−/−animals as detected by immunoblot. (b)In vivoapplication of TSA increases α-tubulin K40 acetylation in control, but not in KO animals. (c) α-tubulin K40 acetylation is undetectable in KO embryos (left panel) and MEFs (right panel). Upon TSA treatment of MEFs the signal of α-tubulin K40 acetylation remained undetectable in KO MEFs. (d) Quantification of (a–c) for representative tissues,n>5. In all images ‘Con’ indicates Atat1fl/flmice and ‘KO’ indicates Atat1−/−mice. ‘DRG’ indicates dorsal root ganglion, ‘kDa’ indicates kilodalton and ‘MEF’ indicates mouse embryonic fibroblasts. Figure 2: Microtubule acetylation in Atat1 −/− mice. ( a ) Absence of detectable α-tubulin K40 acetylation in Atat1 −/− mice as determined by immunoblotting of tissues in adults. Total levels of α-tubulin are not changed in Atat1 −/− animals as detected by immunoblot. ( b ) In vivo application of TSA increases α-tubulin K40 acetylation in control, but not in KO animals. ( c ) α-tubulin K40 acetylation is undetectable in KO embryos (left panel) and MEFs (right panel). Upon TSA treatment of MEFs the signal of α-tubulin K40 acetylation remained undetectable in KO MEFs. ( d ) Quantification of ( a – c ) for representative tissues, n >5. In all images ‘Con’ indicates Atat1 fl/fl mice and ‘KO’ indicates Atat1 −/− mice. ‘DRG’ indicates dorsal root ganglion, ‘kDa’ indicates kilodalton and ‘MEF’ indicates mouse embryonic fibroblasts. Full size image To increase the sensitivity of immunoblot assays and explore the possibility that ongoing deacetylation might mask compensatory mechanisms regulating α-tubulin acetylation in Atat1 −/− animals, we treated mice and fibroblasts with the histone deacetylase inhibitor trichostatin A (TSA). Upon systemic application of TSA in mice we observed a three to fivefold increase in α-tubulin acetylation in tissues from control mice ( Fig. 2b ). In contrast, we were unable to detect an increase in acetylation in any tissue from Atat1 −/− mice, including heart and liver. Similarly, in fibroblasts derived from E12.5 embryos, pretreatment with TSA increased α-tubulin acetylation by fivefold in wild-type cells while no acetylation was detected in cells from Atat1 −/− mice ( Fig. 2c ). Microtubule acetylation has been postulated to have an important role in the nervous system [27] , and it is thus intriguing that Atat1 knockout animals displayed no detectable α-tubulin K40 acetylation in brain, cerebellum and spinal cord. To examine this further, we sought to measure microtubule acetylation in brains from these animals using an alternative pan-acetylated lysine antibody that may detect several other acetylated lysine residues on α- and β-tubulin in vitro [28] . We thus immunoprecipitated brain extracts from Atat1 −/− and Atat1 fl/fl animals with an α-tubulin antibody and immunoblotted eluates with the pan-acetylated lysine antibody. In samples prepared from brain tissue from control animals, we detected a strong signal that was enriched in eluates. Strikingly, however, no signal was detected in Atat1 −/− extracts ( Supplementary Fig. S2 , upper panel). Importantly, we observed no difference in the efficiency of immunoprecipitation in these samples, as immunoblots with the α-tubulin antibody were essentially indistinguishable ( Supplementary Fig. S2 , lower panel). Cellular properties in Atat −/− mice We next investigated α-tubulin acetylation at the subcellular level by examining two cellular structures that have been demonstrated to contain high levels of microtubule acetylation, sperm flagella and neuronal axons [27] , [29] . In sections of testis from control animals we observed strong 6-11b-1 immunofluorescence in the flagellum of sperm and less prominent staining in Sertoli and other cells ( Fig. 3a ). Consistent with our immunoblotting results, we could not detect any α-tubulin acetylation in testis of Atat1 −/− mice, although sperm and their flagella were still evident ( Fig. 3a ). Similarly, in sections of sciatic nerve we observed pronounced α-tubulin acetylation in both large myelinated and small unmyelinated axons of control animals. Sciatic nerve sections from Atat1 −/− mice were, however, completely negative for 6-11b-1 immunoreactivity ( Fig. 3b ). 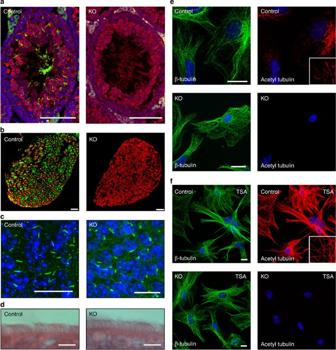Figure 3: Cellular distribution of microtubule acetylation in Atat1−/−mice. (a) Testis sections stained with antibodies against acetylated K40 α-tubulin (green), detyrosinated tubulin (red), and DAPI (blue). Sperm flagella display no detectable K40 α-tubulin acetylation in Atat1−/−mice. Scale bar, 80 μm. (b) Sciatic nerve cross sections stained with antibodies against acetylated K40 α-tubulin (green), and myelin basic protein (red), scale bar, 20 μm. (c) Hippocampal sections stained with DAPI (blue) and an antibody against adenylyl cyclase III (green) to mark cilia, scale bar, 20 μm. (d) H&E staining of oviduct sections showing motile cilia; scale bar, 20 μm. (e) Mouse embryonic fibroblasts stained with antibodies against β-tubulin (green), acetylated K40 α-tubulin (red) and DAPI (blue); scale bar, 20 μm. Inset (size 2.3 μm) shows partially acetylated microtubules. (f) Mouse embryonic fibroblasts stained with the same antibodies as in (e) but after 4 h incubation with Trichostatin A (TSA); scale bar, 20 μm. Inset (size 20 μm shows highly acetylated microtubules). In all images, ‘Control’ indicates Atat1fl/flmice and ‘KO’ indicates Atat1−/−mice. Figure 3: Cellular distribution of microtubule acetylation in Atat1 −/− mice. ( a ) Testis sections stained with antibodies against acetylated K40 α-tubulin (green), detyrosinated tubulin (red), and DAPI (blue). Sperm flagella display no detectable K40 α-tubulin acetylation in Atat1 −/− mice. Scale bar, 80 μm. ( b ) Sciatic nerve cross sections stained with antibodies against acetylated K40 α-tubulin (green), and myelin basic protein (red), scale bar, 20 μm. ( c ) Hippocampal sections stained with DAPI (blue) and an antibody against adenylyl cyclase III (green) to mark cilia, scale bar, 20 μm. ( d ) H&E staining of oviduct sections showing motile cilia; scale bar, 20 μm. ( e ) Mouse embryonic fibroblasts stained with antibodies against β-tubulin (green), acetylated K40 α-tubulin (red) and DAPI (blue); scale bar, 20 μm. Inset (size 2.3 μm) shows partially acetylated microtubules. ( f ) Mouse embryonic fibroblasts stained with the same antibodies as in ( e ) but after 4 h incubation with Trichostatin A (TSA); scale bar, 20 μm. Inset (size 20 μm shows highly acetylated microtubules). In all images, ‘Control’ indicates Atat1 fl/fl mice and ‘KO’ indicates Atat1 −/− mice. Full size image In light of the absence of detectable α-tubulin K40 acetylation in sperm flagella we also examined primary and motile cilia in other cell types. In the hippocampus of Atat1 −/− mice, α-tubulin acetylation was completely absent, however, primary cilia were present at similar densities to control (Atat1 −/− ; 10.3±0.5 cilia per 1,000 μm 2 , Atat1 fl/fl ; 10.5±0.7 cilia per 1,000 μm 2 ) and with comparable morphology and length (Atat1 −/− ; 4±0.4 μm, Atat1 fl/fl ; 3.9±0.2 μm) ( Fig. 3c ). Likewise, in oviduct sections, the number, morphology and length of motile cilia were similar between Atat1 −/− and Atat1 fl/fl mice (Atat1 −/− cilium length; 4.5±0.2 μm, Atat1 fl/fl ; 4.7±0.2 μm, Atat1 −/− cilia density; 15.7±0.6 cilia per 5 μm length of the oviduct, Atat1 fl/fl ; 15.3±0.6 cilia per 5 μm) ( Fig. 3d ). Thus the absence of Atat1 and α-tubulin K40 acetylation does not impact upon the presence or morphological properties of these ciliated organelles. In addition to axons and cilia, microtubule acetylation is also present at lower levels in the cytoplasm of the majority of cells, including embryonic fibroblasts [30] . We therefore derived embryonic fibroblasts from E12.5 embryos and measured α-tubulin acetylation by immunostaining cells with the 6-11b-1 antibody. In agreement with all other experiments, detectable α-tubulin acetylation was absent from cytoplasm of fibroblasts derived from Atat −/− mice, and immunofluorescence was indistinguishable from background levels ( Fig. 3e ). We also treated fibroblasts with the histone deacetylase inhibitor TSA to preclude the possibility that physiological deacetylation was concealing low levels of α-tubulin acetylation. In cells from Atat1 fl/fl mice we observed a pronounced increase in K40 α-tubulin acetylation that was evident on most microtubules within each cell. In contrast, we were unable to detect any immunofluorescence in cells from Atat1 −/− mice ( Fig. 3f ). In embryonic fibroblasts, K40 α-tubulin acetylation is particularly enriched in cilia and basal bodies. We thus serum-starved cells and stained them with an antibody against the cilia marker, AcIII ( Supplementary Fig. S3a,b ). Although Atat1 fl/fl cells displayed strong α-tubulin acetylation in cilia and basal bodies, fibroblasts from Atat1 −/− mice showed no traces of detectable K40 α-tubulin acetylation in these structures. Finally, we sought to determine whether deletion of Atat1 influences the stability of microtubules in embryonic fibroblasts. Post-translational modifications of tubulin such as acetylation accumulate in stable microtubules [31] , however, it is unresolved as to whether acetylation actively stabilizes microtubules [30] , [32] , [33] , [34] , [35] , [36] . As a measure of microtubule stability, we investigated their resistance to nocodazole, a microtubule depolymerizing drug. Following 30 min of incubation with nocodazole, microtubules in fibroblasts from Atat1 fl/fl mice were extensively depolymerized ( Fig. 4a ) and only a few fragments remained ( Fig. 4b ). On the contrary, microtubules in Atat1 −/− fibroblasts were still evident after nocodazole pretreatment ( Fig. 4a ), with obvious fragments of microtubules ( Fig. 4b ). Quantification of these observations revealed that the number of cells that displayed depolymerized microtubules was significantly reduced in fibroblasts from Atat1 −/− mice ( Fig. 4c ), even though these cells contained no detectable K40 α-tubulin acetylation ( Supplementary Fig. S3c ). 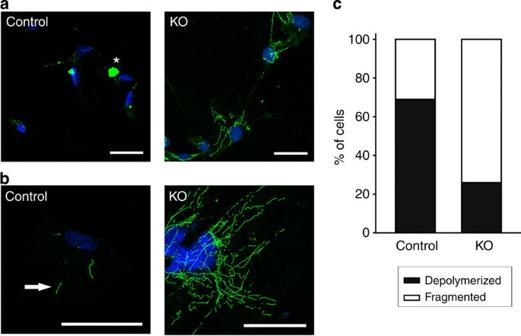Figure 4: Microtubules in Atat1−/−fibroblasts are more resistant to nocodazole-induced depolymerization. Atat1−/−and Atat1fl/flMEFs (labelled ‘KO’ and ‘Control’, respectively), were stained with α-tubulin antibody after a 30-min incubation with nocodazole. (a) Low-magnification images demonstrating that microtubules are extensively depolymerized in control cells (asterisk) while microtubules from Atat1−/−MEFs are resistant. (b) High magnification images showing that fragments of microtubules only occasionally remain in control cells (arrow), while the majority of the microtubule cytoskeleton is present in knockout cells. (c) Quantification of the proportion of fully depolymerized and fragmented microtubules in Atat1−/−and Atat1fl/flMEFs,n=200 cells from three different experiments. Figure 4: Microtubules in Atat1 −/− fibroblasts are more resistant to nocodazole-induced depolymerization. Atat1 −/− and Atat1 fl/fl MEFs (labelled ‘KO’ and ‘Control’, respectively), were stained with α-tubulin antibody after a 30-min incubation with nocodazole. ( a ) Low-magnification images demonstrating that microtubules are extensively depolymerized in control cells (asterisk) while microtubules from Atat1 −/− MEFs are resistant. ( b ) High magnification images showing that fragments of microtubules only occasionally remain in control cells (arrow), while the majority of the microtubule cytoskeleton is present in knockout cells. ( c ) Quantification of the proportion of fully depolymerized and fragmented microtubules in Atat1 −/− and Atat1 fl/fl MEFs, n =200 cells from three different experiments. Full size image Phenotypic analysis of Atat1 −/− mice Despite the apparent absence of microtubule acetylation in Atat1 −/− animals, mice were viable and indistinguishable from control litter mates. To investigate these animals in more detail, we performed a series of phenotypic tests to determine whether the high level of acetylated α-tubulin observed in the brain of wild-type mice is required for normal behaviour, and whether the absence of acetylation impacts upon cell proliferation in the hematopoietic system. We examined neurological behaviour of 8-week-old knockout and control mice (Atat1 −/− body weight; 28.2±1.2 g, Atat1 fl/fl ; 29.8±1.3 g) with a standard battery of tests ( Supplementary Fig. S4 ). At a first-line observation mice of different genotypes seemed indistinguishable. In a more detailed analysis, Atat1 −/− mice displayed normal working memory as measured with a Y maze and normal thermal nociception determined with the hot plate test ( Supplementary Fig. S4a–c ). Muscle strength of all limbs, motor coordination and balance were also unaffected by the loss of Atat1 ( Supplementary Fig. S4d,g ). However, in the open field test, Atat1 −/− mice spent slightly more time in the border area indicating a minor anxiety impairment ( Supplementary Fig. S4e,f ). This finding was supported by a tendency (though not significant) of Atat1 −/− mice to spend less time in the open arms of the elevated plus maze ( Supplementary Fig. S4h,i ). To determine the effects of microtubule acetylation on cell proliferation we examined the haematopoetic system. Inspection of peripheral blood from these animals showed comparable levels of white blood cells in knockout and control animals ( Supplementary Fig. S5a ). The number of red blood cells and haemoglobin levels were also within normal range ( Supplementary Fig. S5b,c ) as was the number of platelets ( Supplementary Fig. S5d ). As we also did not detect any visible developmental defect in Atat1 −/− mice, this indicates that cell proliferation is not grossly affected by deletion of Atat1. Finally, we considered whether progeny number and hence fertility was altered in Atat −/− mice. Heterozygous crossings produced litters with the appropriate Mendelian ratios of homozygote, heterozygote and control pups. Intriguingly, however, we observed a significant decrease in litter size from Atat1 −/− compared with control Atat1 fl/fl crosses (Atat1 −/− ; 7.3±0.5 offspring per cross, Atat1 fl/fl ; 8.9±0.5, P =0.04, Student’s t -test). We investigated the contribution of male fertility to this phenotype by crossing male Atat1 −/− mice with female Atat1 fl/fl mice. Again litter size was significantly reduced (Atat1 −/− males; 7.2±0.5 offspring per cross, Atat1 fl/fl males; 8.9±0.5, P =0.03, Student’s t -test) and the percentage of matings, which resulted in a litter was also lower (Atat1 −/− males 64%, Atat1 fl/fl males 70%). Collating this information revealed that the total number of offspring born from each mating was reduced to 4.6±1 for male Atat1 −/− compared with 7.4±0.9 for male Atat1 fl/fl mice ( P =0.047 from 32 crosses). Thus, deletion of Atat1 impacts upon male mouse fertility. Abnormalities in spermatozoa from Atat1 −/− mice On account of the high level of tubulin acetylation in sperm flagella, and the prominent role of tubulin modifications in cilia [29] , we focused our analysis of mouse fertility on spermatogenesis and axoneme structure and function in Atat −/− mice. We first measured testes and epididymis size, and observed a significant decrease in the weight of these tissues upon Atat1 deletion (Atat1 −/− normalized testis weight; 0.27±0.011% of body weight, Atat1 fl/fl ; 0.32.±0.007%, P =0.003, Student’s t -test. Atat1 −/− normalized epididymis weight; 0.13±0.008%, Atat1 fl/fl ; 0.17.±0.01%, P =0.02, Student’s t -test, all animals were 8 weeks old). In addition, the number of spermatozoa extracted from cauda epididymis was also significantly reduced in Atat1 knockout mice (Atat1 −/− ; 17.5 × 10 6 ±1.3 × 10 6 per ml, Atat1 fl/fl ; 26.9.x10 6 ±1 × 10 6 per ml, P <0.001, Student’s t -test). To examine this further, we undertook a histological examination of testis and observed that H&E stained sections were indistinguishable in Atat1 −/− and Atat1 fl/fl mice ( Fig. 5a ). As a more sensitive measure of cell death in spermatogenesis, we also performed TUNEL staining. TUNEL-positive apoptotic cells were occasionally found in the basal portions of the seminiferous tubules in wild-type mice. Atat1 −/− mice, however, showed increased cell death in seminiferous tubules that was not only present at the basal portion, but throughout the tubules including the luminal side ( Supplementary Fig. S6 ). Thus, Atat1 deletion may have minor effects on the early development of spermatogonia or their maturation into spermatozoa. 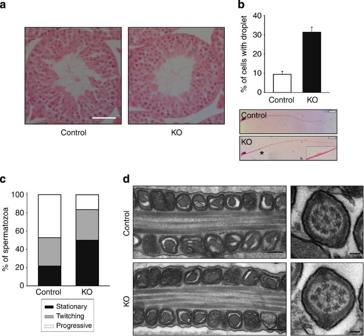Figure 5: Spermatozoa abnormalities in Atat1−/−mice. (a) H&E staining of testis from Atat1−/−and Atat1fl/flmice showing no significant difference between the two genotypes. Scale bar, 50 μm. (b) A larger proportion of Atat1−/−spermatozoa contain a cytoplasmic droplet (n=8 of each genotype). Boxed images show representative examples of spermatozoa. An asterisk marks the position of the cytoplasmic droplet and the inset shows the droplet enlarged. Scale bar, 10 μm. (c) Stacked bar graph showing the percentage of spermatozoa that are stationary, display twitching movement, or have progressive forward motion. Spermatozoa from Atat1−/−mice display less progressive motility. (d) Electron micrographs of sperm flagella from control and Atat1−/−mice. Longitudinal (left panels) and cross sections (right panels) indicate that the 9+2 distribution of microtubules is intact in Atat1−/−mice. Scale bar, 100 nm. In all images, ‘Control’ indicates Atat1fl/flmice and ‘KO’ indicates Atat1−/−mice. Figure 5: Spermatozoa abnormalities in Atat1 −/− mice. ( a ) H&E staining of testis from Atat1 −/− and Atat1 fl/fl mice showing no significant difference between the two genotypes. Scale bar, 50 μm. ( b ) A larger proportion of Atat1 −/− spermatozoa contain a cytoplasmic droplet ( n =8 of each genotype). Boxed images show representative examples of spermatozoa. An asterisk marks the position of the cytoplasmic droplet and the inset shows the droplet enlarged. Scale bar, 10 μm. ( c ) Stacked bar graph showing the percentage of spermatozoa that are stationary, display twitching movement, or have progressive forward motion. Spermatozoa from Atat1 −/− mice display less progressive motility. ( d ) Electron micrographs of sperm flagella from control and Atat1 −/− mice. Longitudinal (left panels) and cross sections (right panels) indicate that the 9+2 distribution of microtubules is intact in Atat1 −/− mice. Scale bar, 100 nm. In all images, ‘Control’ indicates Atat1 fl/fl mice and ‘KO’ indicates Atat1 −/− mice. Full size image We next assessed morphological characteristics of mature spermatozoa isolated from cauda epididymis and observed striking differences in their structure. Concomitant with high levels of tubulin acetylation in the flagella of wild-type sperm, these structures were often disrupted in Atat1 −/− mice and characterized by the presence of a cytoplasmic droplet attached to the annulus of the tail ( Fig. 5b , Atat1 −/− ; 31.34±2.62%, Atat1 fl/fl ; 7.79±1.53%, P <0.00001, Student’s t -test). Cytoplasmic droplets are associated with the impaired maturation of sperm and have been implicated in the process of cytoplasm exclusion and flagellum growth [37] . Although cytoplasmic droplets were occasionally present in spermatozoa from control animals, their occurrence was dramatically increased in sperm from Atat1 −/− mice ( Fig. 5b ). Moreover, flagella length was also significantly decreased in spermatozoa from Atat1 knockout mice, especially in those cells with a cytoplasmic droplet (Atat1 −/− without cytoplasmic droplet; 99.99±0.72 μm, Atat1 −/− with cytoplasmic droplet; 97.94±0.94 μm, Atat1 fl/fl ; 106.01±0.52 μm, P <0.001, Student’s t -test). To determine whether these morphological defects impact upon the function of spermatozoa we investigated sperm motility. Spermatozoa extracted from Atat1 knockout mice displayed significantly lower motility than control sperm. This was evident as a reduction in the number of sperm showing progressive motion, while proportions of stationary cells displaying twitching movement were similar ( Fig. 5c ). We characterized sperm motility further by measuring flagella beat properties. Beat lateral amplitude was reduced in Atat1 knockout mice (Atat1 −/− ; 22.85±1.1 μm, Atat1 fl/fl ; 27.44±0.9 μm, P =0.003, Student’s t -test) as was curvilinear velocity (Atat1 −/− 266.5±6.0 μm s −1 , Atat1 fl/fl 291.11±7.6 μm s −1 , P =0.02, Student’s t -test) indicating that αTAT1 is required for normal flagella motion in spermatozoa. Finally, we examined electron micrographs of sperm flagella from sections of cauda epididymis to determine whether Atat1 deficiency influences the ultrastructural organization of sperm axonemes. Motile cilia possess a characteristic 9+2 organization of axoneme microtubules consisting of 9 outer microtubule doublets and 2 central single microtubules [38] , and this organization has been shown to be disrupted in the absence of other tubulin modifications such as polyglutamylation [3] . In sperm flagella of αTAT1, knockout mice we observed a normal 9+2 distribution ( Fig. 5d ), indicating that αTAT1 and microtubule acetylation exert their effects on flagella structure and function via another mechanism. Here we have examined the consequence of genetic ablation of Atat1 on microtubule acetylation and mouse physiology in vivo . We demonstrate that K40 α-tubulin acetylation is essentially undetectable in Atat1 −/− mice suggesting that αTAT1 is the major mammalian K40 α-tubulin acetyltransferase. Mice are viable and display no major deficits in development, behaviour or adult homeostasis. We did, however, observe a decrease in progeny number from male homozygote Atat1 knockout mice, and deficiencies in the morphology and motility of sperm. As α-tubulin acetylation is particularly enriched in the flagella of sperm, these data suggest that Atat1 may have a role in flagellar function. We were unable to detect acetylated K40 immunoreactivity in Atat1 −/− mice across multiple tissues from adult and embryonic mice as well as in cells derived from these mice. Similarly, treatment of mice or cells with the histone deacetylase inhibitor to block endogenous α-tubulin deacetylation did not unmask any low level acetylation present in Atat1 −/− mice. Thus, in contrast to an earlier report that α-tubulin acetylation persists in zebrafish cilia upon depletion of the Atat1 orthologue mec17 (ref. 17) [17] , our data suggest that mec17 may have not been fully depleted in zebrafish, and that in mice, αTAT1 is likely the major α-tubulin acetyltransferase in both cilia and cytoplasm. Several other candidate acetyltransferases have also been implicated in α-tubulin acetylation, including ARD1-NAT1 (ref. 13) [13] , ELP3 (ref. 14) [14] and GCN5 (ref. 16) [16] . The lack of detectable K40 α-tubulin acetylation in αTAT1 −/− mice reported here indicates that these other enzymes are not able to rescue deficiency of αTAT1, and therefore probably do not acetylate α-tubulin directly in vivo . They may, however, have a role in regulating the expression or activity of αTAT1 and exert their effects on microtubule acetylation indirectly. Despite the apparent absence of α-tubulin acetylation in Atat1 −/− mice, we did not observe any gross defects in the development or homeostasis of these mice. Similarly we could not detect any deficits in cellular structures, which normally express high levels of acetylated α-tubulin, such as axons or primary and motile cilia. This is in broad agreement with previous studies demonstrating that both Chlamydomonas and Tetrahymena have no observable phenotype upon genetic manipulation of native α-tubulin to a non-acetylable form in these organisms [39] , [40] . Moreover, disruption of the α-tubulin deacetylase HDAC6 in mouse results in hyperacetylation of α-tubulin, but does not affect ES cell proliferation or differentiation [41] , or produce substantial phenotypes in mice [30] . Collectively, our data indicate that cells and organisms are able to tolerate considerable shifts in the degree of tubulin acetylation. Intriguingly, we did observe that deletion of Atat1 renders microtubules more resistant to depolymerization in cultured fibroblasts. As nocodazole prevents microtubule growth, but does not perturb existing microtubules, our data show that there are more long-lived (stable) microtubules in KO cells. In support of these findings, we have previously reported that small interfering RNA-mediated depletion of αTAT1 increases microtubule stability and reduces microtubule dynamics [36] . Together these data imply that although acetylated α-tubulin accumulates in stable microtubules [31] , it is not required to actively stabilize microtubules. Indeed, it is likely that αTAT1 has additional roles at microtubules beyond its acetyltransferase function that may serve to regulate dynamic instability and other properties of microtubules [36] , [42] . It is perhaps surprising that Atat1 knockout mice displayed only minor differences in neurological behaviour. α-tubulin acetylation has been suggested to influence kinesin-mediated transport [10] , and increase sensitivity of microtubules to severing in neuronal axons [43] , although these effects may be more dependent upon other tubulin modifications such as tyrosination [44] , [45] and polyglutamylation [46] . Migration and maturation of cortical neurons during development have also been reported to be dependent upon tubulin acetylation [14] , [47] , and depletion of mec17 in zebrafish leads to substantial neurological deficits [17] . We performed behavioural analysis on 8-week-old naïve mice and found only a very mild anxiety phenotype in the open field test. It is possible that further phenotypes only become apparent in older mice or after challenge such as that resulting from disease or pathology. It is, however, clear from our analysis that Atat1 −/− mice represent a powerful tool with which to examine the function of microtubule acetylation in vivo , and in depth analysis of these mice in appropriate models may uncover novel phenotypes. We observed a decrease in litter size from homozygote crosses of Atat1 −/− mice. We reasoned that this may have its basis in altered fertility because we detected no developmental defects in knockout mice and heterozygote crosses produced appropriate Mendelian ratios of Atat1 −/− progeny. We focused our analysis on the male reproductive system as testis has one of the highest levels of microtubule acetylation in control mice. Accordingly, we observed that similar decreases in litter size were also apparent from male Atat1 −/− to female Atat1 fl/fl crosses. We found minor differences in the number of sperm produced by Atat1 −/− mice and more prominent effects on their morphology and motility. Of note, these deficits did not arise from gross structural abnormalities of axoneme organization as has been demonstrated for other tubulin modifications such as polyglutamylation [3] . Rather, we speculate that subtle differences in microtubule function such as intraflagellar transport may account for the shorter flagella in Atat1 −/− mice and subsequent deficits in motility [48] . In summary, we demonstrate that Atat1 is essential for microtubule acetylation in vivo in the mouse. We observed no major deficits in the development or physiology of these mice, however, animals were sub-fertile and displayed abnormal sperm morphology and motility. Atat1 −/− mice thus represent the first in vivo mammalian model for α-tubulin acetylation deficiency and as such could be a valuable tool for exploring the role of this modification in pathology and disease. Generation of the Atat1 null allele The Atat1 targeting strategy was designed to allow Cre-mediated excision of the first six exons of the Atat1 gene that code for the putative acetyltransferase domain of αTAT1. The Atat1 gene-targeting vector ( pDTA-Atat1 ) contained a lox P site 5′ of exon 1, a neomycin resistance ( neo r ) gene flanked with two frt sites, and a lox P site ( neo r -frt2-lox P cassette) located 3′ of exon 6. The targeting construct was transfected into A9 ES cells (A. Wutz, manuscript in preparation). Southern blotting of individual ES cell clones was used to identify homologous recombinants. Positive clones were injected into 8-cell stage embryos to generate mice heterozygous for the targeted allele. Mice were first crossed with FLP-expressing transgenic mice to remove the frt flanked neo r cassette and then to deleter -Cre mice. These genetic manipulations resulted in the generation of Atat1 LoxP alleles (Fl allele), and Atat1 null alleles, respectively. All analysis was performed on mice that did not carry the FLPeR or Del-Cre alleles. Mouse genotype was verified by PCR using primers CCTCTCCCACTATTGTCTCTCATTA (forward for wild-type and LoxP ( fl ) allele), GTATGCCCTTGATGGTGTGTCCCTG (forward for the null allele) and CCTGGAGATGGGTGCATATAAAC (reverse for all). The presence of the Neo cassette (targeted allele) was verified using the forward primer TCCTCCAGCGCGGGGATCTCATG together with the previously mentioned reverse primer. The presence of the FLP transgene was determined with the following primers; CCCATTCCATGCGGGGTATCG and GCATCTGGGAGATCACTGAG . The presence of Cre recombinase was checked with primers GCACTGATTTCGACCAGGTT and GAGTCATCCTTAGCGCCGTA . Mice were bred and maintained at the EMBL Mouse Biology Unit, Monterotondo, in accordance with Italian legislation (Art. 9, 27. Jan 1992, no 116) under licence from the Italian Ministry of Health. Atat1 conditional alleles have been deposited in the European Mutant Mouse Archive ( www.emmanet.org ). Biochemistry and immunohistochemistry All experiments, except Fig. 2c and Fig. 3e , were performed on tissue from 8-week-old mice. Mice were killed by cervical dislocation before the tissues were harvested. For the TSA-induced microtubule acetylation test, animals were injected intraperitoneally with 10 mg kg −1 of Trichostatin A (9950, Cell Signaling) and killed 1 h later. For western blotting, all tissues were homogenized and lysed in buffer containing 150 mM NaCl and 1% Triton X-100. Ten microgram of lysates were used for gel electrophoresis. Western blotting was performed with the following primary antibodies: anti-α-tubulin (T5168, Sigma), anti-acetlylated-α-tubulin (T7451, Sigma), anti-actin (MAB1501, Chemicon), anti-pan-acetylated lysine (AB3879, Chemicon) and the following secondary antibodies: anti-mouse-HRP linked (NA931V, GE Healthcare) and anti-rabbit-HRP linked (NA934V, GE Healthcare). Detection of western blots was performed using the ECL Western blot detection reagent (RPN2106, GE Healthcare). Immunoprecipitation was performed overnight in lysis buffer with the anti-α-tubulin antibody and G protein sepharose beads (17-0618-01, GE Healthcare). Subsequently, proteins were eluted after three washings performed in the same lysis buffer. For histology, oviducts were fixed in 4% paraformaldehyde immediately after dissection, while for the testes and sperm from cauda epididymis modified Davidson’s fluid (2% formaldehyde, 35% EtOH, 10% acetic acid) was used. The tissues were subsequently embedded in paraffin, sectioned and stained with hematoxylin and eosin. Images were taken on a Leica DM 6000B microscope. Sperm morphological parameters were quantified using ImageJ. To detect apoptotic cells in PFA-fixed testes we used the DeadEnd Fluorimetric TUNEL System (TB235, Promega) following the manufacturer’s instructions. Immunostainings of brain, testes and sciatic nerves was also performed on paraffin sections after fixation with PFA. Following rehydration, antigen retrieval was performed with 10 mM sodium citrate (pH 6) at boiling temperature for 10 min. Subsequently, sections were permeabilized (0.3% Triton X-100), blocked (5% goat serum) and stained with anti-acetylated-α-tubulin, anti-myelin basic protein (MAB386, Chemicon), anti-detyrosinated-α-tubulin (AB3201, Millipore), anti-β-tubulin(2146S, Cell Signaling) or anti-adenylyl cyclase III (sc588, Santa Cruz Biotechnology). Samples were examined on a Leica SP5 confocal microscope using a × 20 objective. Processing of images, quantification of fluorescent signal and cilia length quantification were performed using ImageJ. Immunocytochemistry was performed on E 12.5 mouse embryonic fibroblasts (MEFs, passage 2), as previously described [49] . Microtubules were stained using anti-α-tubulin (T5168, Sigma), anti-β-tubulin (2146S, Cell Signaling), and anti-acetylated-α-tubulin (T7451, Sigma) antibodies. For cilia staining, MEFs were serum-starved in Optimem for 48 h before the fixation. For nocodazole-caused microtubule depolymerization test, MEFs were incubated in 10 μM nocodazole (M1404, Sigma) for 30 min before fixation. For the TSA treatment cells were incubated for 4 h with 5 μM TSA (9950, Cell Signaling) before harvesting. All cells were imaged at the Leica SP5 confocal microscope using × 40 and × 63 objectives. The images were processed using ImageJ. Sperm analysis Caudae epididymes from Atat1 fl/fl and Atat1 −/− mice were dissected and aliquots of sperm suspension were used for counting as previously described [50] . Sperm was incubated and analysed in DMEM supplemented with 10% FBS, 75 mg l −1 penicillin, 50 mg l −1 streptomycin, 0.01 mM EDTA, 0.23 mM sodium pyruvate. Sperm motility assays were performed 1 h after dissection on an Axiovert 200 microscope (Zeiss), recording at 25 frames per second. Sperm curvilinear velocity was measured using ImageJ and computer-assisted sperm analyser software, CASA [51] . Beat amplitude was measured using the BeatAnalysis Toolkit [52] . Conventional electron microscopy Caudae epididymes were fixed with a mixture of 2% (w/v) PFA, 2% (w/v) glutaraldehyde (TAAB) in 0.1 M sodium cacodylate buffer (Agar), pH 7.4, post-fixed with 1% (w/v) OsO 4 supplemented with 1.5% (w/v) potassium Ferrocyanide, dehydrated in Ethanol and infiltrated with propylene oxide (Agar)/epon (Agar) (1:1) followed by Epon embedding. Ultrathin sections were cut with an Ultracut S microtome (Leica), counter-stained with Lead Citrate and monitored with a transmission electron microscope (TEM) Jeol 1010. Representative images were obtained using a Gatan MSC 791 CCD camera (Gatan). Behavioural and haematological analysis Behavioural tests were performed on 8-week-old male mice (body weight indicated earlier). All the tests were carried out according to standard procedures described by Eumorphia. Briefly, the Y maze was used to test working memory by detecting the entry into alternating arms of the maze. Alternations are determined as successive entries into each of the three arms as on overlapping triplet sets. Arm exit is defined when all four paws have left the length of the arm. Spontaneous alternation preference is defined as the ratio of actual to possible alternations × 100 and was used as the measure of working memory. Latency to exit the starting arm of the Y maze was scored as an index of emotionality. The hot plate was used to test nociceptive responses to high temperatures. The temperature of the hot plate was set to 55 °C and the latency to the first withdrawal was measured. The grip strength test was used to assess muscle strength of combined forelimbs-hind limbs. A Bioseb grip strength meter apparatus was used. The RotaRod test was used to measure the latency it takes for a mouse to fall off the rod that is rotating under continuous acceleration (from 4 to 40 r.p.m.). An average of four independent trials per mouse was calculated. The open field test was used to assess ambulation in mice as a measurable output of a combination of anxiety and exploratory drive. Locomotor drive of tested animals was comparable to those in the home cage. Elevated plus maze test was used to test the anxiety behaviour. Analysis of peripheral blood was performed using the HV2729 HV950FS Hemavet Unit, following the manufacturer’s instructions. Eight-week-old male mice were used. Statistical analysis Statistical significance was determined using the Student’s t -test. All values are expressed as mean±s.e.m. How to cite this article: Kalebic, N. et al . αTAT1 is the major α-tubulin acetyltransferase in mice. Nat. Commun. 4:1962 doi: 10.1038/ncomms2962 (2013).